Molecular switches from benzene derivatives adsorbed on metal surfaces Transient precursor states are often experimentally observed for molecules adsorbing on surfaces. However, such precursor states are typically rather short-lived, quickly yielding to more stable adsorption configurations. Here we employ first-principles calculations to systematically explore the interaction mechanism for benzene derivatives on metal surfaces, enabling us to selectively tune the stability and the barrier between two metastable adsorption states. In particular, in the case of the tetrachloropyrazine molecule, two equally stable adsorption states are identified with a moderate and conceivably reversible barrier between them. We address the feasibility of experimentally detecting the predicted bistable behaviour and discuss its potential usefulness in a molecular switch. Molecular-scale electronic and optical components are deemed to have an important role in the rapidly evolving information technologies, as well as new energy materials such as photovoltaic solar cells [1] , [2] , [3] , [4] , [5] . In particular, molecules that can be reversibly switched between two or more stable states show great promise for data storage and logical components [3] , [6] , [7] . Tremendous efforts were undertaken to trigger the function of materials at the molecular level, and some promising molecular switches have already been proposed in the literature [8] , [9] , [10] , [11] , [12] , [13] , [14] . Prominent examples of molecular switches include the cis-trans isomerization reaction of azobenzene and its derivatives on surfaces [8] , [9] , [10] , [11] , [12] , as well as the hydrogen tautomerization reaction of the naphthalocyanine molecule [6] , [14] . Recently, Bazarnik et al . [15] reported that by trapping molecules in a physisorption well, direct photo-switching of a dye molecule on metallic surfaces becomes possible. External stimuli such as tunnelling current or light are most frequently used to transform molecules from one state to another. The basic requirements for a molecular switch, that is, bistability and reversibility, can be (partially) achieved through the above mentioned designs. However, many challenges remain in the field of molecular switches, and several complementary designs are currently under investigation [7] , [16] , [17] . The so-called precursor state is traditionally a transient state to chemisorption, into which molecules are trapped before they are strongly bound to the surface [18] . The existence of a precursor state was first proposed by Taylor and Langmuir [19] , then a theoretical model was developed by Kisliuk [20] to interpret the experimental molecular sticking probability as a function of surface coverage. It was not until 1998 that this mobile and transient state was directly observed by means of variable-temperature scanning tunnelling microscopy (STM) for benzene on a (7 × 7) Si(111) surface [21] . From the point of view of modelling, we note that correctly predicting the coexistence of precursor and chemisorption states is a challenge for density-functional theory (DFT), due to the well-known fact that the accurate description of ever-present van der Waals (vdW) interactions is a difficult task for commonly used functionals, especially when studying hybrid organic/inorganic systems. In this Communication, first-principles calculations are used to predict a novel type of bistable system, obtained by controlling the stability and activation barrier between a chemically bound state (the ‘on’ state) and a physically bound (precursor) state (the ‘off’ state) for benzene derivatives adsorbed on a metal surface. The nomenclature of the on and off states refers to the similarity of the operation of the proposed molecular switch to the conventional push-button switches used in many home appliances. We employ DFT calculations including vdW interactions and collective substrate response effects, which allow us to extend beyond the traditional notion of the short-lived precursor state. We demonstrate that the chemical diversity of rigid benzene derivatives offers sufficient flexibility for the design of bistable and potentially reversible molecular switches. Demonstration of bistability for tetrachloropyrazine We first demonstrate the proposed bistability concept for the tetrachloropyrazine (C 4 N 2 Cl 4 ) molecule adsorbed on the Pt(111) surface, which is represented by a six-layer slab with a (4 × 4) unit cell. Our calculations were carried out using the recently developed PBE+vdW surf method [22] (PBE stands for Perdew–Burke–Ernzerhof, see Methods section for computational details), which allows quantitative treatment of both weakly and strongly adsorbed molecules on metal surfaces [22] , [23] , [24] , [25] , [26] . In contrast to conventional adsorption potential-energy curves where only one prominent equilibrium state occurs, the C 4 N 2 Cl 4 /Pt(111) binding curve in Fig. 1a clearly shows the coexistence of two stable states at different adsorption heights, both of them showing essentially equal stability with an adsorption energy of about 1 eV. The off state originating around 3.2 Å is predominantly attributed to vdW interactions, whereas the on state located at 2.1 Å originates from the concerted effect of covalency and vdW bonding [23] , [27] . In fact, the vdW forces have a qualitative impact on the adsorption process, that is, without including vdW interactions there is no binding between C 4 N 2 Cl 4 and Pt(111) for both on and off states. 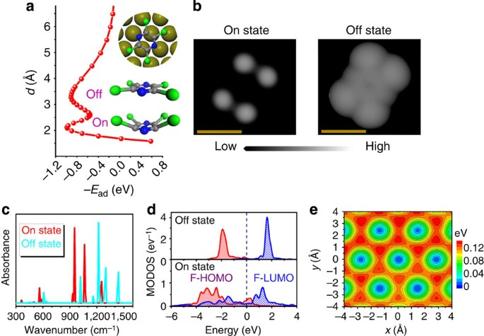Figure 1: Bistable behaviour of tetrachloropyrazine on Pt. (a) Adsorption energy −Ead(xaxis) as a function of the adsorption heightd(yaxis) for tetrachloropyrazine (C4N2Cl4) adsorbed on the Pt(111) surface at the most stable bridge site, with an angle of 30° between the C–N and Pt–Pt bonds (the so-called ‘bridge-30°’ adsorption site; see inset plot). Two stable ground states at differentdare clearly represented in the binding curve, with almost equal stability and a moderate activation barrier between the two states. (b) Constant-current scanning tunnelling microscopy (STM) simulation using the Tersoff–Hamann approximation for C4N2Cl4on the Pt(111) surface at a positive bias voltage of 40 mV. The difference between the two STM images is mainly attributed to the planar (off state) and distorted (on state) structures of the adsorbate. (c) Calculated infrared spectra of C4N2Cl4/Pt(111). Formation of covalent bonds between the adsorbate and the substrate results in a red-shift of the vibrational spectra. (d) Molecular orbital density of states (MODOS) of C4N2Cl4on Pt(111). The former highest occupied molecular orbital (F-HOMO) and former lowest unoccupied molecular orbital (F-LUMO) remain unperturbed in the off state, whereas they strongly overlap in the on state. (e) Contour plot of the potential-energy surface for the C4N2Cl4molecule on the Pt(111) surface in the off state (withd=3.14 Å). (b) Scale bar, 0.5 nm. For more details on the methodology refer to the Methods section. Figure 1: Bistable behaviour of tetrachloropyrazine on Pt. ( a ) Adsorption energy − E ad ( x axis) as a function of the adsorption height d ( y axis) for tetrachloropyrazine (C 4 N 2 Cl 4 ) adsorbed on the Pt(111) surface at the most stable bridge site, with an angle of 30° between the C–N and Pt–Pt bonds (the so-called ‘bridge-30°’ adsorption site; see inset plot). Two stable ground states at different d are clearly represented in the binding curve, with almost equal stability and a moderate activation barrier between the two states. ( b ) Constant-current scanning tunnelling microscopy (STM) simulation using the Tersoff–Hamann approximation for C 4 N 2 Cl 4 on the Pt(111) surface at a positive bias voltage of 40 mV. The difference between the two STM images is mainly attributed to the planar (off state) and distorted (on state) structures of the adsorbate. ( c ) Calculated infrared spectra of C 4 N 2 Cl 4 /Pt(111). Formation of covalent bonds between the adsorbate and the substrate results in a red-shift of the vibrational spectra. ( d ) Molecular orbital density of states (MODOS) of C 4 N 2 Cl 4 on Pt(111). The former highest occupied molecular orbital (F-HOMO) and former lowest unoccupied molecular orbital (F-LUMO) remain unperturbed in the off state, whereas they strongly overlap in the on state. ( e ) Contour plot of the potential-energy surface for the C 4 N 2 Cl 4 molecule on the Pt(111) surface in the off state (with d =3.14 Å). ( b ) Scale bar, 0.5 nm. For more details on the methodology refer to the Methods section. Full size image It is notable from the binding curve that the activation barrier to shift the C 4 N 2 Cl 4 molecule between the off and on states is significantly lower than the barrier for desorption. We determined the structure of the transition state between the two states (see Fig. 2 , inset) using the linear/quadratic synchronous transit method [28] , as implemented in the CASTEP code [29] . The magnitude of the corresponding activation barrier (~0.35 eV) is almost identical to the barrier height deduced from the binding curve (0.36 eV; Fig. 2c ). To assess the impact of the DFT self-interaction error on the activation barrier, the Heyd–Scuseria–Ernzerhof (HSE) hybrid functional [30] , in conjunction with the vdW correction (referred to as HSE+vdW surf ), was employed to recalculate the barriers for C 4 N 2 Cl 4 /Pt(111). Our calculations show that the PBE+vdW surf method gives a very similar barrier compared with the HSE+vdW surf method (0.35 versus 0.31 eV). Dragging the molecule back in the opposite direction, that is, from the on state to the off state, does not lead to hysteresis effects in the C 4 N 2 Cl 4 /Pt(111) system. Furthermore, even for the physisorbed off state of the C 4 N 2 Cl 4 molecule, we find a lateral diffusion barrier of 120 meV on the Pt(111) surface (see Fig. 1e ), which would trap the molecule at a particular adsorption site up to a temperature of ~40–50 K. This stability is also confirmed by ab initio molecular dynamics (AIMD) simulations: during a 10 ps AIMD run at 50 K for this system, we did not observe any changes of the adsorption position, suggesting sufficiently long residence time of C 4 N 2 Cl 4 on Pt(111). 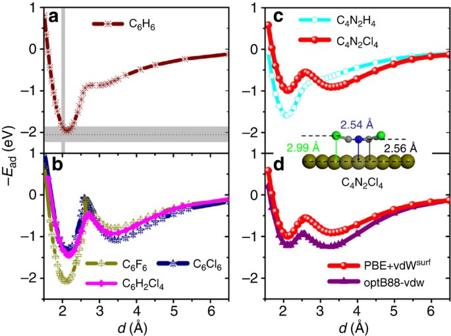Figure 2: Generality of the bistable behaviour for benzene derivatives. (a) Adsorption energy for benzene (C6H6) adsorbed on the Pt(111) surface at the most stable bridge-30° site as a function of distancedfrom the surface. The grey intervals indicate the experimental binding distance based on a low-energy electron diffraction (LEED) analysis45and adsorption energies determined from microcalorimetry measurements36. (b) The binding energy curves for hexafluorobenzene (C6F6), hexachlorobenzene (C6Cl6) and 1,2,4,5-tetrachlorobenzene (C6H2Cl4) on Pt(111). (c) Two additional curves for tetrachloropyrazine (C4N2Cl4) and pyrazine (C4N2H4) on Pt(111). The inset shows the structure of the transition state for the C4N2Cl4molecule. (d) Comparison of the binding energy curves from the PBE+vdWsurfand optB88-vdW methods for the C4N2Cl4/Pt(111) system. For each structure, we fixed thezcoordinates of the carbon backbone and the Pt atoms in the bottom four layers of the six-layer surface model. The adsorption heightdcorresponds to the perpendicular C–Pt distance, which is evaluated relative to the position of the unrelaxed top metal layer. Figure 2: Generality of the bistable behaviour for benzene derivatives. ( a ) Adsorption energy for benzene (C 6 H 6 ) adsorbed on the Pt(111) surface at the most stable bridge-30° site as a function of distance d from the surface. The grey intervals indicate the experimental binding distance based on a low-energy electron diffraction (LEED) analysis [45] and adsorption energies determined from microcalorimetry measurements [36] . ( b ) The binding energy curves for hexafluorobenzene (C 6 F 6 ), hexachlorobenzene (C 6 Cl 6 ) and 1,2,4,5-tetrachlorobenzene (C 6 H 2 Cl 4 ) on Pt(111). ( c ) Two additional curves for tetrachloropyrazine (C 4 N 2 Cl 4 ) and pyrazine (C 4 N 2 H 4 ) on Pt(111). The inset shows the structure of the transition state for the C 4 N 2 Cl 4 molecule. ( d ) Comparison of the binding energy curves from the PBE+vdW surf and optB88-vdW methods for the C 4 N 2 Cl 4 /Pt(111) system. For each structure, we fixed the z coordinates of the carbon backbone and the Pt atoms in the bottom four layers of the six-layer surface model. The adsorption height d corresponds to the perpendicular C–Pt distance, which is evaluated relative to the position of the unrelaxed top metal layer. Full size image We have also compared the PBE+vdW surf binding energy curve with that obtained by the non-local optB88-vdW functional for C 4 N 2 Cl 4 /Pt(111). The optB88-vdW functional [31] , as implemented in the Vienna ab initio simulation package (VASP) [32] , is a modified version of the non-local vdW-density functional [33] . As shown in Fig. 2d , the same qualitative trends are found when using the optB88-vdW method, although overall optB88-vdW gives a somewhat stronger binding compared with the PBE+vdW surf method. The activation barrier between the on and off states is in even better quantitative agreement (0.3–0.4 eV) from both the vdW-inclusive methods. Feasibility of detecting the bistable behaviour A variety of experimental techniques could potentially be used to identify and differentiate between the two states of the tetrachloropyrazine molecule. We first verify the conformational changes by calculating STM images using the Tersoff–Hamann approximation [34] . A small bias voltage of 40 mV was applied to the C 4 N 2 Cl 4 ‘samples’ at on and off states, mapping out the image at constant current. Already here one can unambiguously distinguish the different nature of bonding in the two states. The complete molecular conformation is discernible in the off state (see Fig. 1b ), because C 4 N 2 Cl 4 is flat-lying above the Pt(111) surface with almost zero distortion. However, four bright spots corresponding to the Cl atoms are observed in STM images for each molecule in the on state. This difference stems from the molecular deformation induced on C 4 N 2 Cl 4 forming covalent bonds to the Pt(111) surface. Clear differences can also be observed in the computed infrared vibrational spectra. As shown in Fig. 1c , the on state exhibits a significant red-shift in the infrared frequencies relative to the physisorbed off state. This is rationalized by the fact that formation of the C–Pt and N–Pt covalent bonds weakens the bonding within the molecule. The different electronic properties in the two states are also visible in the computed photoemission spectra. The former HOMO and LUMO (F-HOMO and F-LUMO, respectively) orbitals were calculated by projecting the total density of states of the full system onto the HOMO and LUMO orbitals of the free molecule using the same geometry of the molecule adsorbed on the surface [35] . As illustrated in Fig. 1d , the F-HOMO and F-LUMO significantly broaden on covalent bonding at Pt(111), whereas in the off state both frontier orbitals are only slightly affected relative to those of the free molecule. Analysis of the projected orbital occupations indicates that in the on state there are 1.60 and 0.82 electrons in the F-HOMO and F-LUMO orbitals, respectively. This suggests significant orbital overlap and hybridization between the molecular and surface wavefunctions. In contrast, negligible charge transfer occurs in the off state (1.94 and 0.07 electrons in F-HOMO and F-LUMO, respectively), which confirms the predominant physisorption character of the bonding in this case. Generality of the bistable behaviour To confirm that the proposed bistability concept is a rather general phenomenon, the adsorption energy curves were computed for the C 6 H 6 , C 6 F 6 , C 6 H 2 Cl 4 and C 6 Cl 6 molecules on the Pt(111) surface employing a (4 × 4) unit cell. As shown in Fig. 2a , an incipient precursor state can already be observed for benzene adsorption at 3.1 Å from the Pt(111) surface (similar results have also been found for benzene in a smaller (3 × 3) unit cell [23] ). In fact, Ihm et al . [36] have observed a precursor state in their sticking-coefficient measurements for benzene on Pt(111), although distinguishing between extrinsic and intrinsic precursor states is difficult from these measurements alone. The halogenation of benzene is the most straightforward way to stabilize the precursor state. As illustrated in Fig. 2b , the physisorption strength in the off state increases considerably when the H atoms in benzene are substituted by more polarizable F and Cl atoms (0.78 and 1.05 eV for C 6 F 6 and C 6 Cl 6 on Pt(111), respectively). Owing to the larger vdW radius of the Cl atoms, the C 6 Cl 6 molecule adsorbs at a larger distance from the Pt(111) surface in the off state compared with C 6 F 6 and C 6 H 6 . In the on state, however, the C–Pt covalent bonds largely determine the adsorption height and lead to the same distance for C 6 H 6 , C 6 F 6 , C 6 Cl 6 and C 6 H 2 Cl 4 (2.1 Å; Fig. 2b ). In this case, the vdW interactions stabilize both weakly and strongly bound states [23] , [27] , whereas the vdW energy for C 6 F 6 /Pt(111) is greater than that for C 6 H 6 /Pt(111) (1.27 versus 1.12 eV). Despite the fact that the contribution of vdW energy to the stabilization of C 6 Cl 6 /Pt(111) is 0.5 eV larger than that of C 6 F 6 /Pt(111), in the on state C 6 Cl 6 shows significantly weaker binding to Pt(111) than in the case of C 6 F 6 . In fact, the PBE functional [37] predicts a completely repulsive interaction for C 6 Cl 6 on the Pt(111) surface, whereas C 6 F 6 is already exothermically bound on Pt(111) when using PBE without vdW interactions. Our results demonstrate that on chlorination of benzene, the chemisorption strength to the Pt(111) surface is reduced, whereas the physisorption strength increases. This leads to an adsorption energy curve with two minima having almost equal stability for C 6 Cl 6 . However, the barrier for switching is rather high in this case, comparable in magnitude to the adsorption energy. In contrast to C 6 Cl 6 , our choice of the tetrachloropyrazine molecule leads to the most desirable features: two states with equal stability and a moderate switching barrier between them. The observed bistability phenomenon can be generalized to a wide range of molecules ( cf. Table 1 ). As exemplified by the adsorption of C 6 Cl 6 , C 6 H 2 Cl 4 and C 6 H 4 Cl 2 on the Pt(111) surface, the relative stabilities between the on and off states can be controlled by adjusting the polarizability of the molecule. In addition, larger molecules (for example, C 14 Cl 10 , C 10 Cl 8 and C 10 F 8 ) possess more valence electrons that can be polarized and thus strengthen the vdW bonding. In fact, several interesting trends are noticeable on analysing the computed adsorption energies of the on and off states. As illustrated in Fig. 3 , the reduction of the number of carbon atoms in benzene derivatives considerably destabilizes the on state, whereas increasing the number of chlorine atoms leads to the stabilization of the off state. The two states turn out to have essentially equal stability when there are four C and four Cl atoms in the molecule, providing a rationale for the ‘optimal’ choice of the C 4 N 2 Cl 4 molecule. It is interesting to note that the bistable behaviour is still present when using the F- and Br-containing molecules ( cf. Table 1 ). The peripheral atoms (H, F and Cl) in the C 6 H 6 , C 6 F 6 and C 6 Cl 6 molecules are bent out of the carbon-ring plane in the on state. As they break the aromaticity of the ring, such distortions are expected to be much more costly than in the pyrazine units, such as C 4 N 2 F 4 , C 4 N 2 Cl 4 and C 4 N 2 Br 4 . Table 1 Adsorption of benzene derivatives on Pt. 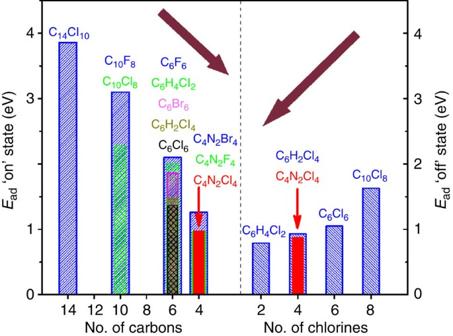Figure 3: Summary of adsorption energies of the two states. Adsorption energyEad(eV) in the on (left panel) and off (right panel) states, respectively, as a function of the number of carbon and chlorine atoms in each molecule adsorbed on the Pt(111) surface. The adsorption energy in the on state decreases with decreasing number of carbon atoms, whereas the adsorption energy in the off state increases with an increase in chlorine atoms. The tetrachloropyrazine (C4N2Cl4) molecule has roughly the same stability in the two states (indicated by red arrows). Full size table Figure 3: Summary of adsorption energies of the two states. Adsorption energy E ad (eV) in the on (left panel) and off (right panel) states, respectively, as a function of the number of carbon and chlorine atoms in each molecule adsorbed on the Pt(111) surface. The adsorption energy in the on state decreases with decreasing number of carbon atoms, whereas the adsorption energy in the off state increases with an increase in chlorine atoms. The tetrachloropyrazine (C 4 N 2 Cl 4 ) molecule has roughly the same stability in the two states (indicated by red arrows). Full size image The substrate surface can also alter the balance between the two states. As shown in Table 2 , for tetrachloropyrazine adsorption on the Cu(111), Ag(111) and Au(111) surfaces, only one adsorption minimum takes place at a typical physisorption height of ~3 Å. This is because coinage metals possess an almost full d -band, which minimizes the chemisorption interaction between the adsorbate and the substrate. In contrast, only a chemisorbed state is identified for the adsorption of tetrachloropyrazine on the Rh(111) surface. Two adsorption minima have been found on full relaxation of the tetrachloropyrazine molecule on the Pd(111), Ir(111) and Pt(111) surfaces ( cf. Table 2 ). Therefore, both the molecule and the substrate are key factors in the design of bistable adsorbed molecules. Table 2 Adsorption of tetrachloropyrazine on metal surfaces. Full size table The proposed bistability mechanism is clearly a general phenomenon that exists for a variety of molecules and metallic surfaces. In particular, the tetrachloropyrazine molecule is bistable and was predicted to be functional up to a temperature of ~40–50 K. We also performed 10 ps AIMD simulation at a higher temperature of 150 K, starting with C 4 N 2 Cl 4 physisorbed in the off state. We found that sliding along the surface plane is the dominant effect at this temperature. This indicates that sliding is the process with the lowest barrier when starting from the off state. To realize a reversible single-molecule switch with higher operating temperatures, one could tailor different functional groups in a molecule and look for molecules adsorbing slightly closer (for example, 0.1 or 0.2 Å) to metal surfaces in the physisorbed off state. In this case, the molecule remains in a stable physisorbed state, but with a more corrugated potential-energy surface that would prevent surface diffusion at elevated temperatures. Apart from the force-induced switching, other switching mechanisms, for example, applying voltage pulses to the molecule using an STM tip, should be tested. Encouraging results have been reported very recently by Huang et al . [13] , showing that the molecular-switching direction can be changed by applying a voltage pulse, either positive or negative, through the STM tip to the target molecule. In summary, using first-principles calculations, we designed a bistable organic/inorganic system based on switching between two vertical ground-state configurations of a small molecule adsorbed on a metal surface. The vdW energy dramatically stabilizes the physisorption state, extending the conventional notion of the metastable and short-lived precursor state. The structure, vibrational and electronic properties are remarkably different in the so-called on and off states, allowing for the two states to be distinguished. Theoretical methods We used density-functional theory with van der Waals interactions (PBE+vdW surf method [22] ), as implemented in the FHI-aims all-electron code [38] . The PBE+vdW surf method extends pairwise vdW approaches to modelling of adsorbates on surfaces by a synergetic combination of the PBE+vdW method [39] for intermolecular interactions with the Lifshitz–Zaremba–Kohn theory [40] , [41] for the non-local Coulomb screening within the bulk. The PBE+vdW surf method [22] includes the collective many-body response (screening) of the substrate electrons in the determination of the C 6 coefficients and vdW radii, going beyond the pairwise description. It has already been shown that the PBE+vdW surf method yields excellent agreement with experiments for a variety of atoms and molecules adsorbed on metal surfaces, including the rare-gas atoms, benzene, 2-pyrrolidone, naphthalene and 3,4,9,10-perylene-tetracarboxylic acid dianhydride adsorbed on several close-packed transition-metal surfaces [22] , [23] , [24] , [25] . The relativistic effects were treated by using scaled zeroth-order regular approximation [42] . We employed the ‘tight’ settings for integration grids and standard numerical atom-centered orbitals basis sets in FHI-aims code. We used the FHI-aims ‘tier2’ basis set for light elements such as H, C, N and F, and ‘tier1’ for Cl, Br and transition metals Cu, Ag, Au, Rh, Pd, Ir and Pt. These settings ensure meV total-energy accuracy from the electrostatic and integration grid settings used. A convergence criterion of 10 −2 eV Å −1 for the maximum final force was used for structural relaxations and a convergence criteria of 10 −5 electrons per unit volume for the charge density and 10 −4 eV for the total energy of the system was utilized for all computations. In slab calculations, we used a 6 × 6 × 1 Monkhorst–Pack mesh for the sampling of the Brillouin zone of the (4 × 4) surface. In the optB88-vdW calculations, core electrons were replaced by PBE-based projector augmented wave potentials [43] in the VASP code [32] , whereas valence electrons were expanded in plane-waves with a cut-off energy of 500 eV. A Monkhorst–Pack mesh with 4 × 4 × 1 k -point sampling was used. In addition, we calculated the STM images in the framework of the Tersoff–Hamann approximation [34] , by including Kohn–Sham eigenstates between the Fermi level and a given voltage. Infrared vibrational spectra were calculated by a second derivative of the energy from the numerical change of the forces arising from small finite displacements. Six finite displacements were applied to each of the atoms with a value of 0.005 Å. Adsorption models and convergence tests In our calculations metal surfaces were modelled by six-layer slabs. For geometry optimizations, the molecule and the two uppermost metal layers were allowed to fully relax, and the metal atoms of the bottommost four layers were constrained at their bulk positions. Different slabs were separated by 20 Å of vacuum. Our recent work [44] has systematically assessed the reliability of results for benzene adsorption on Pt(111) by comparison with adsorption energies obtained by microcalorimetry measurements of Campbell's group [36] . For benzene on Pt(111) with a (4 × 4) unit cell, the adsorption energy computed by the PBE+vdW surf (2.18 eV) is within the uncertainty of microcalorimetry measurements in the limit of zero coverage (1.84–2.25 eV) [36] . Further increase of the unit cell to (5 × 5) only leads to 20 meV difference in adsorption energy and thus a (4 × 4) cell used in the current work is sufficient to exclude the intermolecular interactions between periodic images of the molecules. The spin moment of the entire system and the magnetic states of Pt(111) remain unchanged on inclusion of spin polarization in our calculations. How to cite this article: Liu, W. et al . Molecular switches from benzene derivatives adsorbed on metal surfaces. Nat. Commun. 4:2569 doi: 10.1038/ncomms3569 (2013).